Fluid signal suppression characteristics of 3D-FLAIR with a T2 selective inversion pulse in the skull base 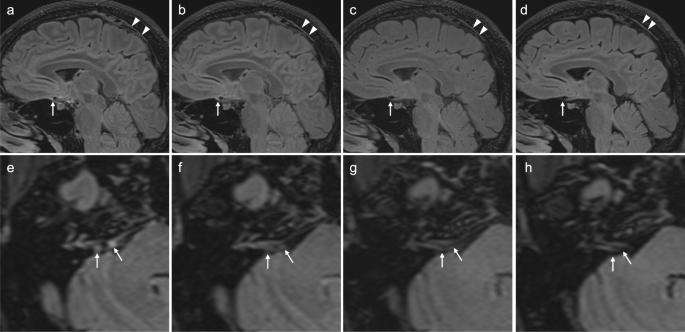Fig. 1: 3D-FLAIR images obtained in a healthy male volunteer in his 40 s. 3D-FLAIR image obtained with T2-selective inversion pulse (a,e), that with T2-preparation pulses (b,f), that with conventional inversion pulse (c,g), and that with conventional inversion using longer repetition time of 8000 msec (d,h). MR imaging was performed at Siemens 3 Tesla using a 32-channel array head coil similar to that used in the article in ref.3. MR imaging parameters are comparable to that in the article by Albayram et al.; TR/TE/TI: 5000/387/1700 for (a–c), and (e,f), 8000/387/2370 for (d,h), 0.9 mm resolution, using fat suppression. Sagittal images (a–d) and axial images (e–h) are presented. A similar contrast between gray/white matter as in the images in the article by Albayram et al. was achieved in (a,e), (b,f), and (d,h). Linear high signal along superior sagittal sinus, which is presumed to be lymphatic tissue, is visualized in all images (arrow heads ina–d). Linear high signal (arrow) presumed to be lymphatic tissue anterior to the pituitary gland is visualized most prominently in (a) as in the images in the article by Albayram et al., less prominently in (b) and far less prominently in (c,d). Nodular high signal areas (arrows) near the orifice of internal auditory canal which are presumed to be lymphatic tissue are visualized most prominently in (e), far less prominently in (f) and not in (g,h). Judging from these volunteer images, the images in the article by Albayram et al. is thought to be obtained with 3D-FLAIR using a T2-selective inversion pulse. 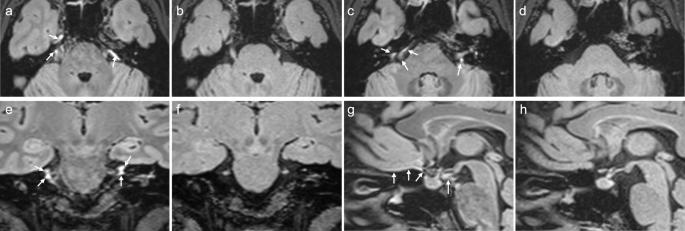Fig. 2: Comparison of 3D-FLAIR imaging with a T2-selective inversion pulse to that obtained with a conventional inversion pulse in a healthy female volunteer in her 40 s. MR imaging was performed at Siemens 3 Tesla using a 32-channel array head coil similar to that used in the article by Albayram et al.3. The scan parameters are also comparable to those used in the article by Albayram et al. In the 3D-FLAIR imaging with a T2-selective inversion pulse (a,c,e,g), similar contrast between gray/white matter is achieved as in the images shown in the article by Albayram et al. even with the same repetition time of 5000 msec. In 3D-FLAIR imaging with a conventional inversion pulse (b,d,f,h), less contrast between gray/white matter is provided than observed in the images of the article by Albayram et al. using the same repetition time of 5000 msec. High signal intensity, which corresponds to the areas presumed to be lymphatic tissues in Fig. 4 of the article by Albayram et al. (arrows ina,c,e,g) is only visible in the 3D-FLAIR images obtained with a T2-selective inversion pulse. The MR images in this work were obtained with a 3 Tesla scanner (Skyra, Siemens Healthineers, Erlangen, Germany) using 32-channel head coils. Four types of 3D-FLAIR images were obtained using the following parameters: The echo time of 387 msec was used for all four types of 3D-FLAIR. The repetition time (TR) of 5000 msec was used for three kinds of 3D-FLAIR data sets, and the TR of 8000 msec was used for the other 3D-FLAIR dataset. Conventional inversion recovery (IR) pulse, T2-selective IR pulse, and T2-preparation pulse were applied to three types of 3D-FLAIR data sets with TR of 5000 msec, respectively. For 3D-FLAIR with TR of 8000 msec, the conventional IR pulse was used. The inversion time for three types of 3D-FLAIR data sets with TR of 5000 msec was 1700 msec. For the 3D-FLAIR with TR of 8000 msec, the inversion time was set to 2370 msec to null the CSF signal. Research involving human participants and/or animals This manuscript contains human volunteers’ image data. The Medical Ethics Board, Nagoya University Graduate School of Medicine, approved this study (2021-0309 22949). Reporting summary Further information on research design is available in the Nature Portfolio Reporting Summary linked to this article.